Admixture facilitates genetic adaptations to high altitude in Tibet Admixture is recognized as a widespread feature of human populations, renewing interest in the possibility that genetic exchange can facilitate adaptations to new environments. Studies of Tibetans revealed candidates for high-altitude adaptations in the EGLN1 and EPAS1 genes, associated with lower haemoglobin concentration. However, the history of these variants or that of Tibetans remains poorly understood. Here we analyse genotype data for the Nepalese Sherpa, and find that Tibetans are a mixture of ancestral populations related to the Sherpa and Han Chinese. EGLN1 and EPAS1 genes show a striking enrichment of high-altitude ancestry in the Tibetan genome, indicating that migrants from low altitude acquired adaptive alleles from the highlanders. Accordingly, the Sherpa and Tibetans share adaptive haemoglobin traits. This admixture-mediated adaptation shares important features with adaptive introgression. Therefore, we identify a novel mechanism, beyond selection on new mutations or on standing variation, through which populations can adapt to local environments. The environments and indigenous populations of high altitude ( ⩾ 2,500 m in altitude) are an ideal study system for understanding the genetic basis of adaptive traits [1] . Low barometric pressure and consequent physiological hypoxia constitute a strong selective pressure [2] , [3] , [4] , [5] , which is unavoidable and invariant across individuals at a given altitude because it cannot be influenced by behavioural or cultural practices [1] . A distinctive set of physiological traits found in Tibetan highlanders, including unelevated haemoglobin concentrations up to 4,000 m altitude, are clearly linked to O 2 delivery [3] . In Tibetans, variants in the EGLN1 (egl nine homologue 1) and EPAS1 (endothelial PAS-domain containing protein 1) genes harbour signals of adaptive allele frequency divergence relative to low-altitude East Asian populations as well as association signals with haemoglobin concentration [3] , [4] , [5] . These genes are major components of the HIF (hypoxia-inducible factor) pathway, which senses and reacts to changes in O 2 supply [6] . Despite these recent insights, the evolutionary history of these adaptive alleles remains poorly understood. The genetic history of East Asian populations includes complex patterns of ancient admixture [7] , [8] , [9] , but little is known about the genetic relationship of Tibetans with other East Asian populations. The dramatic growth of low-altitude East Asian populations in the past 10,000–30,000 years inferred based on genome sequence data [10] , [11] is likely to have created intense demographic pressure, possibly leading to expansion into the Tibetan plateau and genetic exchange with resident populations. This mixing of populations from different local environments, in turn, would create the potential for transfer of alleles advantageous at high altitude to the gene pool of migrants. To resolve the genetic history of Tibetans and of their adaptation to high-altitude, we obtained genetic and phenotypic data for a sample of 69 Sherpa, a population famous for their superb performance in mountaineering and an example of successful adaptation to high-altitude environments. All sampled individuals were born and raised at ⩾ 3,000 m altitude in the Himalayas. Genotypes of 96 unrelated Tibetan individuals from three previous studies [3] , [4] , [12] were also analysed. These individuals were sampled in three different high-altitude regions of the plateau: the Tibet Autonomous Region (near Lhasa) [12] , Yunnan [3] and Qinghai [4] provinces in China (3,200–4,350 m altitude). We merged the genotype data of the Sherpa and Tibetans with the International HapMap phase 3 (HapMap3) data set [13] using imputation for non-overlapping variants. For some analyses, this data set was combined with additional genotype data for the following populations: worldwide populations in the HGDP (Human Genome Diversity Panel) [9] , [14] , Indian and Central Asian populations [15] and two Siberian populations [16] . Here we show that Tibetans are the admixed descendants of ancestral populations related to contemporary Sherpa and Han Chinese. We also show that high-altitude adaptive variants originated in an ancestral population (represented by present-day Sherpa) and that they preferentially propagated in the Tibetan gene pool after admixture. Our results provide a clear example of transfer of adaptive alleles between human populations, which is supported by ancestry-based tests, population genetic signatures of local adaptations and by adaptive phenotype data. The admixture origin of Tibetans We first conducted descriptive analyses to assess the population structure of the Sherpa and Tibetans within the context of other Asians. Interestingly, the Sherpa and Tibetans form a major axis of genetic variation in principal component analysis (PCA) [17] , in which Tibetans are located between the Sherpa and other East Asians (PC2 in Fig. 1a ). Although the pattern observed in the PCA plot can result from several demographic processes (for example, strong genetic drift in the Sherpa), it is also consistent with a history of admixture in Tibetans between ancestral populations closely related to the contemporary Sherpa and low-altitude East Asians. Unsupervised clustering analysis using ADMIXTURE [18] also infers Tibetans as a mixture of two genetic components: one is highly enriched in the Sherpa (but rare in lowlander populations) and will be referred to as the ‘high-altitude component’ and the other in low-altitude East Asians and will be referred to as the ‘low-altitude component’ ( Fig. 1b ). The inclusion of a broader range of Asian populations shows that the high-altitude component is not due to shared ancestry with South or Central Asians ( Supplementary Figs 1–3 ). 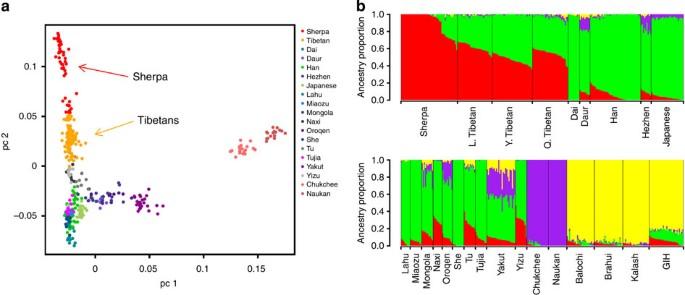Figure 1: The genetic structure of Sherpa and Tibetans relative to other East Asian populations. (a) PCA of Sherpa (49 unrelated individuals), Tibetans (n=96), maritime Chukchee (n=19), Naukan Yup’ik (n=16) and East Asian populations from the HGDP (n=210). PC1 and PC2 explain 2.5 and 1.2% of total variation, respectively. (b) ADMIXTURE analysis withK=4. Red and green colours represent the high-altitude and low-altitude components, respectively. Yellow and purple ancestries are mainly present in the Indian–Pakistani and Siberian populations, respectively. L. Tibetan=Lhasa Tibetan12(n=30); Y. Tibetan=Yunnan Tibetan3(n=35); Q. Tibetan=Qinghai Tibetan4(n=31); GIH=HapMap3 GIH (Gujarati Indians from Houston, Texas, USA;n=30). Balochi (n=24), Brahui (n=25) and Kalash (n=23) are from the HGDP. The Sherpa also show evidence of admixture with East Asians ( Supplementary Table 1 ) and marked inter-individual variation in ancestry proportions, but they are unique in harbouring individuals with 100% inferred high-altitude component ( Fig. 1 , Supplementary Figs 1 and 2 ). 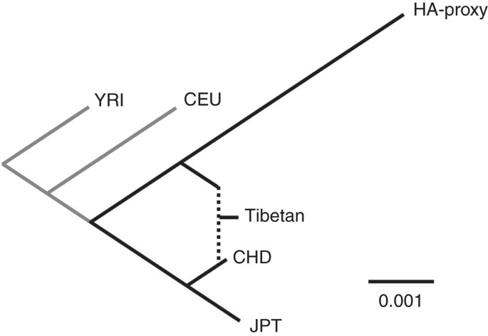Figure 2: Tibetans as a mixture of the HA-proxy and Han Chinese-related ancestral populations in the scaffold tree. Grey branches are not drawn to proportion. The scale bar represents 0.001 in the drift unit. YRI=Yoruba in Ibadan, Nigeria; CEU=Utah residents with Northern and Western European ancestry from the CEPH collection; CHD=Chinese in Metropolitan Denver, Colorado, USA; JPT=Japanese in Tokyo, Japan. The date of this East Asian admixture into the Sherpa was estimated to be 23.4 generations ago, based on the decay of linkage disequilibrium (LD) [7] (see Methods; Supplementary Figs 4 and 5 , and Supplementary Table 2 ). This date is in close agreement with the historical record of a Sherpa migration out of their ancestral homeland in Eastern Tibet 400–600 years ago to their current place, Solu-Khumbu [19] . In subsequent analyses, we considered the subset of 21 individuals with 100% high-altitude component (referred to as HA-proxy sample; ‘HA’ for high altitude) to be the descendants of an ancient high-altitude population with a broad geographic distribution across the plateau. Taken together, these results strongly suggest that Tibetans are admixed descendants of two populations currently represented by the HA-proxy and low-altitude East Asians (such as Han Chinese), while the Sherpa more recently experienced admixture with nearby East Asian populations, most likely Tibetans ( Supplementary Fig. 5 ). Figure 1: The genetic structure of Sherpa and Tibetans relative to other East Asian populations. ( a ) PCA of Sherpa (49 unrelated individuals), Tibetans ( n =96), maritime Chukchee ( n =19), Naukan Yup’ik ( n =16) and East Asian populations from the HGDP ( n =210). PC1 and PC2 explain 2.5 and 1.2% of total variation, respectively. ( b ) ADMIXTURE analysis with K =4. Red and green colours represent the high-altitude and low-altitude components, respectively. Yellow and purple ancestries are mainly present in the Indian–Pakistani and Siberian populations, respectively. L. Tibetan=Lhasa Tibetan [12] ( n =30); Y. Tibetan=Yunnan Tibetan [3] ( n =35); Q. Tibetan=Qinghai Tibetan [4] ( n =31); GIH=HapMap3 GIH (Gujarati Indians from Houston, Texas, USA; n =30). Balochi ( n =24), Brahui ( n =25) and Kalash ( n =23) are from the HGDP. Full size image Formal tests of admixture give further support to the admixture hypothesis of Tibetan origin. We used the D-test and 3-population (f 3 ) test [9] , both of which exploit the pattern of shared genetic drift from the moments of allele frequency. The D-test asks if a set of four populations fits into a simple bifurcating tree. Under this null, two pairs of populations with non-overlapping drift paths are expected; thus, there is no shared genetic drift and the expectation of the D statistic is zero. Admixture breaks up the bifurcating tree topology and generates an overlap of drift paths, making the D statistic deviate from zero. The 3-population test uses information about the shared genetic drift between a target population and each of two reference populations. Under the null of a bifurcating tree, the shared genetic drift is the drift that occurred on the branch leading to the target population and the f 3 statistic is expected to take a markedly positive value. Therefore, a negative value is strong evidence for a deviation from the null. We used HapMap3 YRI (Yoruba in Ibadan, Nigeria) as the outgroup, CHD (Chinese in Metropolitan Denver, Colorado, USA) as representative of the ancestral low-altitude East Asians, and the HA-proxy sample as representative of the ancestral high-altitude population. D-test results were highly significant for all three Tibetan populations (D=−5.1 to −9.8 s.d. 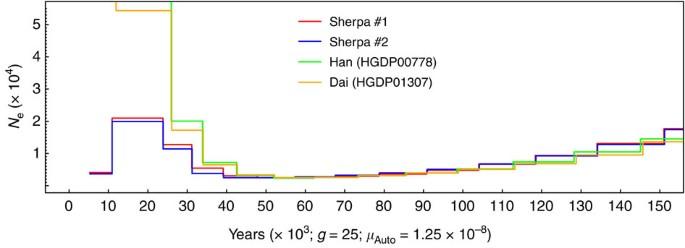Figure 3: Whole-genome sequence based inference on effective population size. The effective population sizes (Ne) of the ancestral high- and low-altitude populations are inferred from whole-genome sequences of two Sherpa and two low-altitude East Asians (a Han and a Dai individual) (g=generation time in year;μAuto=autosomal neutral mutation rate per base per generation). ; see Methods; Supplementary Table 3 ). The 3-population test results were also negative (f 3 =−1.5 to −3.5 s.d. ; see Methods; Supplementary Table 3 ). Tests with the other two HapMap3 East Asian populations, CHB (Han Chinese in Beijing, China) and JPT (Japanese in Tokyo, Japan), showed similar results ( Supplementary Table 3 ). Furthermore, all the Tibetan samples were consistently positioned in the population tree as a mixture of branches leading to the HA-proxy and CHD, using either MixMapper [8] ( Fig. 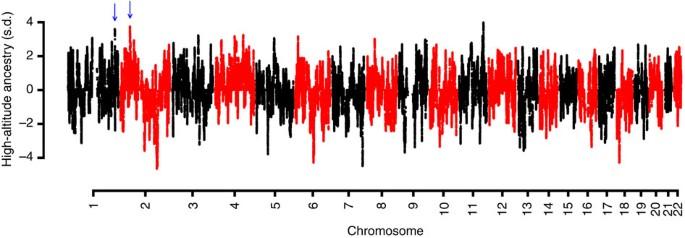Figure 4: The distribution of high-altitude ancestry proportions across the Tibetan genome. Blue arrows mark the positions ofEGLN1(in chromosome 1) andEPAS1(in chromosome 2). 2 and Supplementary Table 4 ) or TreeMix [20] ( Supplementary Fig. 6 and Supplementary Table 5 ). An LD decay method [7] that tests for admixture and estimates the admixture timing did not detect a signal in Tibetans and, hence, could not be used to estimate the admixture timing. This method is known to lose power with increasing time since admixture more quickly than the 3-population test [7] and, possibly, other methods based on genetic drift. Given the significant admixture signals from the 3-population test, the D-test, MixMapper and TreeMix as well as the patterns observed in the ADMIXTURE and PCA plots, we speculate that the results of the LD decay method reflect an old admixture date (see Methods; Supplementary Fig. 7 and Supplementary Table 2 ). Figure 2: Tibetans as a mixture of the HA-proxy and Han Chinese-related ancestral populations in the scaffold tree. Grey branches are not drawn to proportion. The scale bar represents 0.001 in the drift unit. YRI=Yoruba in Ibadan, Nigeria; CEU=Utah residents with Northern and Western European ancestry from the CEPH collection; CHD=Chinese in Metropolitan Denver, Colorado, USA; JPT=Japanese in Tokyo, Japan. Full size image The demography of the ancestral high-altitude population To learn about the genetic history of the ancestral population that contributed to the Tibetan gene pool, we sequenced the genomes of two HA-proxy males to high coverage (27–30x) and inferred the history of population size using the Pairwise Sequentially Markovian Coalescent (PSMC) model [10] . Interestingly, the high-altitude demographic profile begins to diverge from that of Han Chinese and Dai [11] ~40,000 years ago and shows no signature of the dramatic exponential population growth characterizing low-altitude East Asians (see Methods; Fig. 3 ). The same analysis with pairs of X chromosome sequences gives estimates of the split time between the high-altitude and the low-altitude populations of ~20,000 years ago (see Methods; Supplementary Fig. 8 ). These results suggest that the ancestral high-altitude population diverged from other low-altitude East Asians in our sample during the upper Palaeolithic. This is consistent with previous proposals based on archaeological, mitochondrial DNA (mtDNA) and Y chromosome data, pointing to an initial colonization of the Tibetan plateau ~30,000 years ago [21] , [22] . A second, more recent migration to Tibet was proposed based on mtDNA and Y chromosome data [21] , which is consistent not only with our admixture hypothesis but also with archaeological evidence [22] . Figure 3: Whole-genome sequence based inference on effective population size. The effective population sizes ( N e ) of the ancestral high- and low-altitude populations are inferred from whole-genome sequences of two Sherpa and two low-altitude East Asians (a Han and a Dai individual) ( g =generation time in year; μ Auto =autosomal neutral mutation rate per base per generation). Full size image To learn more about the history of the newly detected high-altitude ancestry component, we analysed the HA-proxy samples for admixture with archaic humans, that is, Neanderthal and Denisovan. We tested whether the HA-proxy or Tibetans experienced different levels of admixture with archaic hominins relative to other modern human populations. When projected onto the PC plane defined by the Chimpanzee, Neanderthal and Denisovan genotype data, the HA-proxy and Tibetans clustered with the other HGDP East Asian populations ( Supplementary Fig. 9 ). The D-test results also show that the HA-proxy and Tibetans have Neanderthal ancestry similar to those of Eurasian populations but higher than those of African populations. As all other Eurasian populations, the HA-proxy and Tibetans have Denisovan ancestry lower than that of Papuans ( Supplementary Table 6 ). These results suggest that the history of ancient admixture in the ancestral high-altitude population does not differ substantially from that of other East Asian populations. Selection and association signals in Sherpa and Tibetans At the phenotypic level, the Sherpa, like Tibetans, have unelevated haemoglobin concentration at high altitude [23] ( Supplementary Table 7 ). To ask whether the sharing of this adaptive phenotype is due to shared beneficial alleles, we conducted population genetic and genetic association analyses in our Sherpa data. The SNPs near EGLN1 and EPAS1 with the highest population branch statistic (PBS) [5] in Tibetans also had top PBS values in the HA-proxy (see Methods; Supplementary Table 8 ). We also replicated, in the Sherpa, associations between EPAS1 SNPs and haemoglobin concentration previously reported in Tibetans [3] . Specifically, 19 out of 26 significant SNPs in Tibetans were also associated with haemoglobin levels in the Sherpa (linear mixed model (LMM) P <0.05; N =69), all with the same allelic direction reported in Tibetans (see Methods; Supplementary Table 9 ). This is a significant enrichment in low P -values as only 3 out of 1,000 permutations showed ⩾ 19 SNPs with P <0.05 ( Supplementary Table 10 ). Adaptive excess of high-altitude ancestry in Tibetans These findings indicate that Tibetans share genetic adaptations with the Sherpa despite a substantial amount of gene flow from low-altitude East Asians ( Fig. 1 ), leading to the hypothesis that alleles associated with lower haemoglobin levels preferentially propagated in the admixed gene pool. Consistent with this hypothesis, an analysis of inferred local ancestry of Tibetans using HAPMIX [24] clearly showed that the EGLN1 (3.59 s.d.) and EPAS1 (3.74 s.d.) genes are highly enriched for high-altitude ancestry, representing respectively the second and the third strongest signals of excess high-altitude ancestry in the Tibetan genome (see Methods; Fig. 4 and Supplementary Fig. 10 ). In addition, SNPs with excess high-altitude ancestry are significantly enriched around genes involved in the HIF pathway (Reactome pathways gene set ‘Cellular response to hypoxia’; Supplementary Table 11 ) [25] , even after removing EGLN1 and EPAS1 genes (see Methods; Supplementary Table 12 ). We also modelled Tibetan allele frequencies as a linear combination of those of the 11 HapMap3 populations and the HA-proxy (see Methods) [26] . SNPs with large residuals in the linear model are likely to be a departure from the average admixture proportion in the Tibetan genome. Using multiple regression (MR) and the linear coefficients estimated using all SNPs, we found that SNPs in and around EGLN1 and EPAS1 SNPs had extremely large residuals, further supporting the idea that alleles in these genes disproportionately increased in frequency in Tibetans after admixture ( Supplementary Figs 11 and 12 ). Figure 4: The distribution of high-altitude ancestry proportions across the Tibetan genome. Blue arrows mark the positions of EGLN1 (in chromosome 1) and EPAS1 (in chromosome 2). Full size image Interestingly, the SNP with the largest high-altitude ancestry proportion in the Tibetan genome (rs1003081; Fig. 4 ) lies <1 kb away from a candidate gene for hypoxia adaptations, hypoxia upregulated protein 1 ( HYOU1 ), which encodes a molecular chaperone induced in the endoplasmic reticulum under hypoxic condition [27] , [28] ( Supplementary Fig. 13 ). The same SNP is also a cis expression quantitative trait locus for another nearby candidate gene, hydroxymethylbilane synthase ( HMBS ; Supplementary Fig. 13 ), in liver [29] and monocytes [30] . This gene encodes the third enzyme in the haem biosynthesis pathway [31] ; therefore, variation in this gene could have a direct effect on haemoglobin concentration. We tested SNPs in this peak of high-altitude ancestry for an association with haemoglobin levels in the 69 Sherpa and found that 19 of 64 SNPs have P <0.05 (LMM, Supplementary Table 13 ). Only 12 out of 1,000 permutations have ⩾ 19 SNPs with P <0.05, indicating a significant enrichment of low association P -values in this region ( Supplementary Table 14 ). A local excess of high-altitude ancestry might also be generated under a simple branching model of population history without admixture if selection acted in parallel in the Sherpa and Tibetans on a variant that predated their split. However, given the strong evidence for admixture described above, the excess of high-altitude ancestry at known adaptive loci argues for selection on these variants in the admixed population. Our results show that adaptations can be facilitated by admixture with locally adapted resident populations. Gene flow has been appreciated as a source of adaptive alleles by theoretical population geneticists for a long time, but few cases in animals have been documented at the empirical level and several of them have only partial support in the data [32] , [33] , [34] , [35] , [36] , [37] . Here we reported a case of adaptation facilitated by gene flow between modern human populations that is supported by ancestry-based analysis, phenotypic data and population genetic evidence. Given the prevalence of admixture in humans, our findings suggest that this mode of adaptation may be common and that further examples may be found in other populations, for example, Asian Indians [38] , Europeans [39] and Sub-Saharan Africans [40] , which originated from the mixture of ancestral gene pools with different local adaptations. Interestingly, the evolutionary dynamics of these admixture-driven adaptations closely resembles that of adaptively introgressed alleles across a species boundary. Our demographic model for high-altitude populations suggests a much older split between high- and lowlanders compared with a previous model based on exome sequence data [5] . As a consequence, we estimated selection coefficients of 0.0004–0.0023 for the variants in EGLN1 and EPAS1 gene regions in the HA-proxy sample (see Methods; Supplementary Table 15 ). In contrast to a previous proposal [5] , our estimates are an order of magnitude smaller than those for lactose tolerance alleles in Europe and Africa [41] . However, all these estimates depend on many model assumptions and are typically associated with large uncertainties; therefore, further analyses are necessary to obtain accurate estimates of the selection coefficient. The acquisition of adaptive variants through gene flow adds a new dimension to the ongoing debate on the relative importance of selective sweeps and polygenic adaptations in human evolution [42] . Unlike selective sweeps and polygenic adaptations, gene flow can introduce a suite of adaptive alleles that evolved in concert and that segregate at appreciable frequencies in the admixed population. Finally, our findings highlight the importance of sampling unique branches of the human population tree, such as the Sherpa, to detect admixture events and to elucidate the history of human adaptations. Study subjects Demographic, phenotypic and genetic data were collected from 69 high-altitude native Sherpa residing in two villages at 3,800 m in the Khumbu region of Nepal during the summer of 2010 ( Supplementary Table 7 ). The participants were healthy non-smoking men and women, born and raised above 3,000 m altitude, 17–54 years of age, who had not travelled to areas <2,400 m or >5,400 m in the previous 6 months, had normal body mass index, lung function and blood pressure, were not anaemic, did not have fever and were not pregnant. All study participants provided written informed consent. This study was approved by the IRBs at Case Western Reserve University and University of Chicago, by the Oxford Tropical Research Ethics Committee and by the Nepal Health Research Council. Phenotypic data collection Standing height without shoes (GPM Anthropometer, Stuttgart, Switzerland) and weight in light clothing (Pelouze Mechanical Shipping Scale, P114S, Bridgeview, Illinois, USA) were measured to the nearest mm and pound, respectively, according to standard protocol [43] . Blood haemoglobin concentration was measured in duplicate using the cyanmethaemoglobin technique (Hemocue, Angelholm, Switzerland) immediately after venipuncture. Genotype data All the Sherpa samples were genotyped using Illumina HumanOmni1-Quad beadchip in the Genomics Core Facility at Case Western Reserve University. We removed SNPs with call rate <95%, minor allele frequency <5% or with strand-ambiguity. Genetic relatives were inferred from a random set of 2,000 autosomal SNPs using Relpair v2.0.1 (ref. 44 ). Twenty related individuals with closer relationships than first cousins were excluded in subsequent analyses except for the genotype–phenotype association test. We also obtained genotype data of 96 Tibetans from three previous studies, each including 30–35 individuals ( Supplementary Table 16 ) [3] , [4] , [12] . As all three data sets are from different regions of the Tibetan plateau and from different genotyping platforms (Illumina Human1M-Duo v3 for Lhasa Tibetans [12] , Illumina Human610-Quad for Yunnan Tibetans [3] and Affymetrix Genome-wide Human SNP 6.0 for Qinghai Tibetans [4] ), most of the analyses were conducted on the three Tibetan samples separately. To maximize the overlap between data sets, we imputed the Sherpa and the three Tibetan genotype data sets using IMPUTE2 (ref. 45 ) with the HapMap3 data set ( Supplementary Table 17 ) [13] as a reference. Each of four data sets was imputed separately. For each individual and SNP, we called a genotype if it had posterior probability ⩾ 0.9, otherwise, we treated it as missing data. We excluded SNPs with call rate <96.5% in the Sherpa or in any of the three Tibetan samples ( ⩾ 3 missing genotypes in the Sherpa or ⩾ 2 missing genotypes in Tibetans). This process yielded 543,555 SNPs overlapping between the Sherpa, Tibetans and HapMap3 data sets (‘HM3’; n =1,165); before imputation, 80,819 overlapping SNPs were identified. To analyse Sherpa and Tibetan genetic variation in a broader context, we overlapped this data set with each of three additional data sets. First, we overlapped it with data from HGDP [14] and two Siberian populations, Naukan Yup’ik and maritime Chukchee [16] , to obtain 50,464 SNPs with genotype call rate ⩾ 96.5% for all populations in the data set (‘HM3–HGDP’; n =2,138). Second, we overlapped the HM3 data set with HGDP individuals genotyped on Affymetrix Axiom Genome-wide Human Origins 1 array, described by Patterson et al . [9] We obtained 58,756 SNPs (‘HM3-HumanOrigin’; n =2,107) after excluding strand-ambiguous or low-quality SNPs ( ⩾ 2 missing genotypes in any of the 53 HGDP populations). Last, we overlapped the HM3 data set with the genotype data of 14 Asian populations (Thai, Vietnamese, Cambodian, Iban, Buryat, Kyrgyzstani, Nepalese, Pakistani, Andhra Pradesh Brahmins, Andhra Pradesh Madiga, Andhra Pradesh Mala, Tamil Nadu Brahmins, Tamil Nadu Dalit and Irulas) from Xing et al . [15] We obtained 62,541 SNPs after excluding strand-ambiguous or low-quality ( ⩾ 2 missing genotypes in any of the 14 Asian populations) SNPs (‘HM3-Asian’; n =1,418). Analyses of admixture We used EIGENSOFT 4.2 (ref. 17 ) to perform PCA. For unsupervised clustering analysis, we used ADMIXTURE v1.22 (ref. 18 ) with fivefold cross validation to find the optimal number of clusters. When using the HM3-Asian data set for ADMIXTURE analysis, we generated LD-trimmed SNP sets by removing one SNP from each pair of SNPs with r 2 >0.2 in 50 SNP blocks using PLINK v1.07 (ref. 46 ). The D-test and 3-population test were performed as implemented in ADMIXTOOLS v1.1 (ref. 9 ). We used ALDER [7] to date the admixture event using admixture LD decay. To reduce the noise introduced by genetic drift specific to the HA-proxy sample and CHD, we used SNP loadings of a principal component (PC) representing the Sherpa–Tibetan axis of genetic variation as a weight vector instead of allele frequency difference between two reference populations. To obtain this weight vector, we ran a PCA with the Sherpa, Tibetans and HapMap3 CHD (Chinese in Metropolitan Denver, Colorado), CHB (Han Chinese in Beijing, China), JPT (Japanese in Tokyo, Japan) and GIH (Gujarati Indians in Houston, Texas) ( Supplementary Fig. 14 ). SNP loadings of the second PC were used as a weight vector. A bin size of 0.25 centiMorgan (cM) was used for all analyses. When fitting the exponential curve, we excluded SNP pairs within distance bins of ⩽ 0.5 cM to remove those in LD in the ancestral populations. Significance of the estimates was assessed by block jackknifing of one chromosome at a time. Whole-genome sequence analysis Two Sherpa males with 100% high-altitude ancestry component were chosen for 100-bp paired-end whole-genome sequencing using Illumina HiSeq 2000. We followed a standard Illumina TruSeq DNA sample preparation protocol for paired-end sequencing to construct sequencing libraries. Each sample was tagged with a unique adapter sequence. We mixed an equal amount of library DNA from two samples and sequenced the mixed library in a flow cell. After separating raw reads using adapter sequences, we mapped reads onto the human genome reference sequence (hg19) using BWA [47] . We further adjusted the alignment by conducting local realignment around indels and base quality recalibration steps using Genome Analysis Tool Kit [48] . After removing duplicates using Picard, we called consensus genome sequences of each individual using Samtools v0.1.19 (ref. 49) [49] . We applied the Pairwise Sequentially Markovian Coalescent (PSMC) model [10] to autosomal consensus sequence of each sample separately, using the following options: −N15−t15−r5−p ‘2*2+50*1+4+6’. To compare them with low-altitude East Asians, we downloaded the aligned sequence reads (in BAM file format) for a Han Chinese and a Dai individual from Meyer et al . [11] These sequence data were generated using essentially the same protocol as for our sequence data: sequencing libraries were prepared following the standard Illumina TruSeq DNA sample preparation protocol for paired-end sequencing of 101 bp reads and 200–400 bp insert size, sequencing was performed on an Illumina HiSeq 2000, reads were mapped to the human genome reference sequence (hg19) using BWA [47] , and the coverage was 27.7 × and 28.3 × for a Han and a Dai individual, respectively. In addition, to minimize any bias introduced by differences in post-alignment processing, we processed the Han and Dai reads in the same way as we did for the Sherpa samples. To convert the estimates of population parameters into the effective population size ( N e ) and time in year, we used autosomal neutral mutation rate μ Auto =1.25 × 10 −8 per base-pair per generation and 25 years per generation [50] . We also applied the PSMC model to composite diploid X chromosome sequences, composed of two haploid X chromosome sequences from two males. For this analysis, we called the genotypes of X chromosome sequences using the same pipeline applied to the autosomal sequences and called a heterozygote if the haploid genotype calls of two individuals are different at a site. Sites with a missing genotype in either of two individuals were coded as missing data. We ran the PSMC with the options −N25−t15−r5−p ‘6+2*4+3+13*2+3+2*4+6’. Time bins were sliced in a coarser way than those for the autosomal data, considering the lower resolution of X chromosome data. We adjusted the neutral mutation rate for X chromosome ( μ X ) by applying the ratio of male-to-female mutation rate α =2 (ref. 51 ) and the formula μ X = μ Auto × [2(2+ α )]/[3(1+ α )]=1.11 × 10 −8 (ref. 10 ) All raw sequences generated in this study have been deposited into the Sequence Read Archive (NCBI) with the accession numbers SRS520217 and SRS520218. Local ancestry estimation We estimated local ancestry across the genome of three Tibetan samples using HAPMIX [24] , using the 21 HA-proxy and the 21 CHD individuals with the highest proportion of the low-altitude component as the reference populations ( Fig. 1b ). Phased genotypes of CHD individuals were obtained from the HapMap3 website. The Sherpa genotype data were phased by using fastPHASE [52] . We estimated the local ancestry of each of the three Tibetan samples separately, using 50% admixture proportion, 80 generations since admixture and population recombination parameter ρ =600 for both reference populations. To summarize the local ancestry estimates across the three samples, we first individually centred local ancestry estimates by subtracting individual mean local ancestry (MLA). Then, we averaged local ancestry of each SNP across all individuals and standardized these mean values of local ancestry. We repeated this step for each of three Tibetan samples separately. To guard against the effect of genotyping error in the estimated local ancestry, we additionally ran HAPMIX with only half of the SNPs in Tibetans (odd- and even-numbered SNPs, respectively). False local ancestry peaks inferred from genotyping errors at a SNP will disappear in only one of these two sets. Therefore, we defined a penalty for the MLA value of each SNP, where the penalty is the absolute difference between MLAs from the odd-numbered and even-numbered SNP sets. We adjusted the estimated MLA by So, this adjustment reduces the peak height toward zero in proportion to the difference between odd/even SNP sets. If this adjustment changes the sign of MLA, we set MLA to zero. After adjustment, we standardized MLA ( Fig. 4 and Supplementary Fig. 10 ). Gene set enrichment analysis We tested for an enrichment of genes involved in the response to hypoxia in the regions with excess high-altitude ancestry across the Tibetan genome. We focused on the Reactome pathway gene set ‘Cellular response to hypoxia’ (25 genes) and its subset ‘Oxygen-dependent proline hydroxylation of HIF alpha’ (18 genes; Supplementary Table 11 ) [25] . To determine whether there was an excess of SNPs with high high-altitude ancestry in the gene sets, we calculated top 0.5, 1.0 or 5.0 percentile of the high-altitude local ancestry of all SNPs within 10 kb of all genes except for the hypoxia genes. Then, we calculated the proportion of SNPs with higher high-altitude local ancestry than the above percentiles within 10 kb of genes in the gene set of interest. We repeated this process 1,000 times by bootstrapping the whole genome and counted the number of bootstrap replicates for which the proportion of the top high-altitude ancestry SNPs in the hypoxia genes is higher than the corresponding percentile. We repeated the enrichment analysis after removing EGLN1 and EPAS1 genes from the gene set. PBS analysis To detect SNPs showing high divergence of allele frequency in the Sherpa and Tibetans from low-altitude East Asians, we calculated the PBS of each SNP in the HA-proxy and each of three Tibetan samples. To maximize the amount of the genome covered by SNPs, we used a lenient SNP filtering by allowing up to 10% missing genotypes for the HA-proxy and for each of three Tibetan samples, resulting in 879,434 SNPs (‘extended HM3’). We also merged all three Tibetan samples to increase accuracy in allele frequency estimates. We chose HapMap3 CHD and CEU (Utah residents with Northern and Western European ancestry from the CEPH collection) to represent a low-altitude East Asian population and the outgroup, respectively. We followed Weir and Cockerham [53] to calculate pair-wise F ST and Yi et al . [5] to calculate PBS. We retrieved SNPs with the highest rank around EGLN1 and EPAS1 genes (within 300 kb) in Tibetans and checked their ranks in the HA-proxy. All analyses were performed using R v2.15.1 (ref. 54 ). MR analysis To identify SNPs with extreme frequency divergence in Tibetans while taking into account their history of admixture, we used a MR analysis described in Alkorta-Aranburu et al . [26] Briefly, we modelled Tibetan allele frequencies in the extended HM3 data set as a linear combination of those of the 11 HapMap3 populations ( Supplementary Table 17 ) and the HA-proxy. Alleles were polarized based on the global allele frequency. We obtained the standardized and squared residuals (‘MR score’) from the above MR model. We took the rank of each SNP, divided it by the total number of the SNPs and minus log 10 transformed to get the transformed rank. Genetic association with haemoglobin levels in the Sherpa For the EPAS1 gene region on chromosome 2, SNP genotypes in a 5 Mb region were imputed using IMPUTE2 (ref. 45 ) with 1,000 Genomes phase 1 integrated variant set [55] as a reference panel. SNPs with information metric ⩾ 0.9 were chosen for downstream analysis. Twenty-six SNPs passed this threshold among those reported to be associated with haemoglobin concentration in two Tibetan cohorts [3] . For the HYOU1 / HMBS gene region on chromosome 11, we selected the 64 genotyped SNPs with high-altitude ancestry ⩾ 3.7 s.d. ( Supplementary Fig. 13 ). We tested for a genetic association between mean posterior genotype of these SNPs and haemoglobin concentration in all 69 Sherpa individuals. We took relatedness among samples into account through a LMM scheme using GEMMA [56] ( Supplementary Tables 9 and 13 ). Genetic relatedness between individuals was estimated using the genome-wide genotype data. We included sex as a covariate. One thousand permutations of concentration across individuals were performed to test whether the results were significantly enriched for low P -values ( Supplementary Tables 10 and 14 ). Mapping of admixed populations on phylogenetic trees We used MixMapper [8] and TreeMix [20] to infer the ancestral populations contributing to the Tibetan gene pool and the proportion of admixture in a single step. We ran MixMapper with a scaffold tree of five populations (the HA-proxy, HapMap3 YRI, CEU, CHD and JPT) using the HM3 data set. These five populations were chosen to cover major branches of human populations and to reduce computational load. We also ran TreeMix , with each of the three Tibetan populations and the above five populations. We allowed three admixture events for each of these six-population sets. In both MixMapper and TreeMix analyses, we performed 500 bootstrap replicates with 50 SNPs as a block for bootstrap sampling. Archaic human admixture in the Sherpa and Tibetans We ran PCA for Chimpanzee, Neanderthal and Denisovan genotype data (HM3-HumanOrigin data set) and obtained the projection of modern human individuals on these PCs. Population means of PC1 and PC2 were plotted for the 53 HGDP populations, the HA-proxy and three Tibetan samples. We also performed the D-test. The D statistic was calculated for each of ((H 1 , H 2 ), (A, Chimpanzee)) quartets with the HM3-HumanOrigin data set: H 1 =the 53 HGDP populations; H 2 =the HA-proxy/Tibetans; A=Neanderthal or Denisovan. Estimating the selection coefficient Given the sharing of adaptive variants in the EGLN1 and EPAS1 gene regions between Tibetans and the HA-proxy, we estimated selection coefficients of these variants in the HA-proxy because its demography is simpler than that of Tibetans. Here we applied a simple deterministic model of selective sweep with additive genetic effects, using the following formula: We estimated the initial allele frequency ( p 0 ) as the mean allele frequency of the three HapMap3 East Asian populations: CHD, CHB and JPT. The current allele frequency ( p t ) was estimated as the allele frequency of the HA-proxy. We chose eight SNPs (five in EGLN1 and three in EPAS1 region; Supplementary Table 15 ), which have top PBS signals in the HA-proxy and Tibetans and are not in complete LD with each other. Based on our estimate of the split time of 20,000 years, we used 800 generations (with 25 years per generation; Supplementary Fig. 8 ) for the onset of selection ( t ) in the ancestral high-altitude population, assuming that selection began right after the population split. Accession codes : The DNA sequences have been deposited in the NCBI’s Sequence Read Archive under the accession codes SRS520217 and SRS520218 . How to cite this article: Jeong, C. et al . Admixture-facilitated genetic adaptations to high altitude in Tibet. Nat. Commun. 5:3281 doi: 10.1038/ncomms4281 (2014).